Surfactant-enabled epitaxy through control of growth mode with chemical boundary conditions Property coupling at interfaces between active materials is a rich source of functionality, if defect densities are low, interfaces are smooth and the microstructure is featureless. Conventional synthesis techniques generally fail to achieve this when materials have highly dissimilar structure, symmetry and bond type—precisely when the potential for property engineering is most pronounced. Here we present a general synthesis methodology, involving systematic control of the chemical boundary conditions in situ , by which the crystal habit, and thus growth mode, can be actively engineered. In so doing, we establish the capability for layer-by-layer deposition in systems that otherwise default to island formation and grainy morphology. This technique is demonstrated via atomically smooth {111} calcium oxide films on (0001) gallium nitride. The operative surfactant-based mechanism is verified by temperature-dependent predictions from ab initio thermodynamic calculations. Calcium oxide films with smooth morphology exhibit a three order of magnitude enhancement of insulation resistance. Heteroepitaxy is the enabling integration platform for indispensable microelectronic devices including semiconductor quantum wells, superconducting tunnel junctions, solid-state lasers, light-emitting diodes, and extreme-mobility transistors. Heteroepitaxy is also the technique of choice to synthesize artificial crystalline structures that provide access to new effects, including multiferroic exchange biasing, ordered nanostructure evolution, and interfacial nanoelectronics [1] , [2] , [3] . In most cases, these technologies and capabilities are relegated to systems where the end members are isostructural, for example, zincblende–zincblende or perovskite–perovskite. This limitation stems from the seemingly insuperable challenges of preparing semiconductor-grade epitaxial thin films on substrates that are strongly dissimilar in symmetry or bonding character, even when lattice mismatch is very small. We could expect, however, a rich resource of new science and functionalities at ideal epitaxial interfaces between highly dissimilar materials, if they could be created. The opportunities become particularly interesting if we can exploit property coupling between polar semiconductors and materials close to a phase transition or property instability; these include nonlinear dielectrics, non-linear magnets, and/or two-dimensional conductors [4] , [5] , [6] , [7] , [8] . This vision for integration is made possible by introducing a novel synthesis technique that provides access to highly mismatched epitaxial systems that cannot be realized by conventional methods. The method relies on engineering chemical boundary conditions with a vapour phase surfactant, thus stabilizing a specific crystalline habit and enabling layer-by-layer growth. Demonstrated for a simple prototype, this method promises an extension to numerous materials systems with improved performance, and entirely new functional modalities. Precedents for such dramatic impacts on morphology at heterointerfaces are not available. To illustrate the power of this paradigm we consider a particularly challenging prototype: 〈111〉 oriented CaO on [0001]-oriented GaN. Our selection of CaO/GaN is inspired by the need for wide band gap pseudomorphic insulators on Al 1-x Ga x N. Smooth oxide films on GaN provide a parallel platform to LaAlO 3 /SrTiO 3 heterostructres that are of great current interest for nanoelectronic devices based on conducting interfaces. This also is an ideal candidate pair because CaO and other rocksalts exhibit extreme propensity for {001} faceting (from very strong surface energy contrast between the low-index planes) [9] , [10] , [11] , whereas the hexagonal face of GaN promotes a 〈111〉 CaO epitaxial growth orientation. With conventional growth techniques, at only several monolayers thickness, rocksalt films collapse into pyramidal islands with {100} faces [9] , [10] , [11] . This seemingly unavoidable behaviour leads to a grainy morphology and diminished functionality [12] , [13] . The surfactant-assisted method applied currently to CaO can be extended to more complicated systems. A prime example is the cubic perovskites, which will in almost every case encounter the identical roadblock if prepared on wide band gap polar semiconductors. Overcoming this obstacle to film growth with a surfactant creates new integration possibilities, such as BaTiO 3 on Al 1-x Ga x N, thus a new ability to harness the associated functionality. We describe below MBE deposition of CaO in the presence of a water-based surfactant that enables continuous 〈111〉 CaO films grown in a 2D mode. The CaO films retain the step-and-terrace morphology of their parent substrates and demonstrate the ability to engineer growth mode by controlling the chemical boundary conditions. These trends are understood using a quantitative surface-energy-based model that is based on a companion set of temperature-dependent ab-initio thermodynamic calculations. Thermodynamic evaluation To overcome the morphology challenge, we demonstrate a true surfactant methodology where a transient chemical species resident to the growing film surface can alter the relative energetics of different crystallographic faces in situ to growth. The paradigm for surfactant selection is based on creating a monolayer-thick skin of a surface phase that has a low surface energy plane that exhibits sixfold symmetry to match that of (0001) GaN, epitaxial registry to the final film and becomes chemically unstable if incorporated to the film interior. From a crystal chemistry and thermodynamic perspective, Ca(OH) 2 satisfies these criteria and can be prepared by supplying a continuous flux of water vapour that supplies both oxygen for reactive growth and the hydrogen surfactant. In this scenario, an obvious concern is competition between MO and M(OH) 2 deposition particularly because low substrate temperatures (that is, 200 to 500 °C) are needed to limit Ca re-evaporation. The relative free energies of formation for each species can be compared with predict, if a window exists where bulk hydroxide is unstable in the partial pressure range appropriate for MBE. 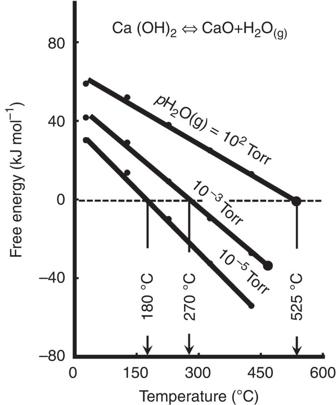Figure 1: Phase diagram for the system Ca(OH)2-CaO-O2. Free energy of the calcium hydroxide decomposition reaction versus temperature at 1 atmosphere, 10−3Torr, and 10−5Torr water partial pressures. Figure 1 shows the temperature- and pressure-dependent equilibrium connecting calcium oxide, calcium hydroxide and water vapour [14] . These data predict the onset of hydroxide decomposition in a temperature and pressure window consistent with reactive growth of CaO, using practical fluxes and growth rates. This calculation assumes bulk equilibrium and predicts that, at a substrate temperature, within this range, one expects only CaO accumulation. However, as reported by Kandel et al ., because the free energy of a finite system is lowered by the presence of surfactant moieties at a surface, we speculate that the temperature at which hydroxide leaves a {111} CaO surface will be higher [15] . Consequently, it is sensible to hypothesize that an ideal temperature for surfactant-assisted growth exists just above the temperature stability maximum for Ca(OH) 2 ; in this region it is likely that a CaO bulk film with a hydrogen-terminated surface is energetically preferred. Figure 1: Phase diagram for the system Ca(OH) 2 -CaO-O 2 . Free energy of the calcium hydroxide decomposition reaction versus temperature at 1 atmosphere, 10 −3 Torr, and 10 −5 Torr water partial pressures. Full size image Film deposition To explore this hypothesis, CaO thin films were grown by oxide MBE onto [0001] oriented Ga-face c + -polar films that exhibit a single and uniform polar orientation [16] . Ca was evaporated from a thermal source while the oxidant was supplied as an ambient of either molecular oxygen or water vapour. These two gas phase constituents provide the comparison of conventional and surfactant-assisted growth. Reflection high energy electron diffraction (RHEED) was used to monitor film deposition. 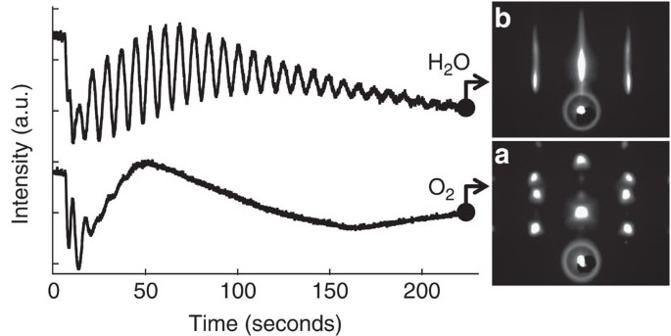Figure 2: RHEED comparison for CaO growth in oxygen and water vapour. RHEED data for 〈111〉 CaO epitaxial films prepared on [0001] GaN. (a) Corresponds to a film grown in molecular oxygen whereas (b) corresponds to a film grown in an equivalent flux of water vapour. All other deposition conditions are identical. The intensity vs. time plots are collected from the specular reflection. Figure 2 shows a RHEED comparison of integrated specular intensity as a function of time during growth and a static RHEED pattern of the CaO terminal surfaces grown in oxygen and water vapour environments, with all other conditions identical. Figure 2: RHEED comparison for CaO growth in oxygen and water vapour. RHEED data for 〈111〉 CaO epitaxial films prepared on [0001] GaN. ( a ) Corresponds to a film grown in molecular oxygen whereas ( b ) corresponds to a film grown in an equivalent flux of water vapour. All other deposition conditions are identical. The intensity vs. time plots are collected from the specular reflection. Full size image In both cases, the substrate is exposed to oxidant, at the deposition temperature, and growth is initiated by opening the Ca source shutter. The RHEED pattern in Figure 2b has a spotty character consistent with electron transmission diffraction along a surface that is rough at the atomic scale. The intensity vs time plot shows a weak initial oscillation, which may be interpreted as the growth of a smooth initial monolayer, and then a rapid transition to island formation and three-dimensional growth. In comparison, Figure 2a shows the same electron diffraction analysis for a CaO film prepared in an equivalent flux of water vapour. In this case, steady RHEED intensity oscillations are observed during the entire process, indicating 2D growth, and the final static RHEED image is streaky, indicating a smooth (though crystallographically imperfect) surface [17] . We note that the oscillation amplitude decays with time. This is consistent with simultaneous growth of multiple layers with time, and a step-bunching transition that occurs for epitaxial growth on vicinal surfaces [18] . The sapphire wafers in this work are nominally on axis, but the growth spirals create surface regions that are effectively miscut. At the early stages of growth in water, the first intensity maximum occurs at a non-integer time interval compared with subsequent periodic maxima. We hypothesize that this results from the reaction of Ca with the existing GaN native oxide (which is 1 ml for GaN exposed to ambient conditions at RT) to create the first CaO monolayer. Similar interactions have been reported by Nozawa et al ., where 1.5 ml of aluminum metal reacted with the GaN native oxide forming a surface mixture of Al-metal and aluminum oxide at 200 °C (ref. 19 ). It is likely that the low sticking coefficient of H 2 O on an oxidized GaN surface promotes this behaviour, that is, the oxygen that terminates the GaN surface is kinetically more available than the oxygen from ambient water. This scenario changes after the first monolayer of CaO because this suface supports rapid dissociative chemisorption of H 2 O (ref. 20 ). To further test this scenario, CaO films were prepared on H-terminated GaN substrates produced by HF-last chemical etching before growth. On these surfaces, the initial non-integer peak is not present. Film characterization To physically confirm film morphology, AFM images were collected from 4.5 nm CaO thin films immediately after deposition. CaO, however, is extremely susceptible to hydroxide formation at room temperature, thus, to protect the samples from water attack, they were capped in situ with four monolayers of Dy 2 O 3 . This Dy 2 O 3 thickness, monitored by RHEED oscillations, was found to be the thinnest coating that provided protection against water attack for several hours. At small thicknesses, dysprosia thin films are stabilized in the hexagonal allotrope, which grows smooth on surfaces with hexagonal symmetry. The dysprosia surfaces are stable for practical periods of time with respect to hydroxylation. 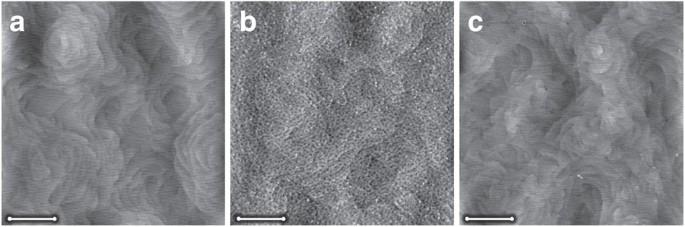Figure 3: Surface topography comparison for CaO films prepared in oxygen and water vapour. (a) GaN starting surface, which is populated by growth spirals with 0.26 nm step heights. These spirals initiate around screw dislocations and are consistent with layer-by-layer growth from a supersaturated MOCVD ambient. (b) 4.5 nm CaO film grown in molecular oxygen. The AFM resolves clearly the grainy nature of the CaO coating and how the fine grains decorate the underlying GaN steps and terraces; the RMS roughness over a 5×5 μm area is 0.5 nm. (c) 4.5 nm CaO film grown with water vapour; all other conditions identical the step and terrace morphology of the GaN is preserved and the RMS roughness over 5×5 μm is 0.3 nm. Figure 3 shows the comparison of the starting GaN surface, and capped CaO films grown with and without a water surfactant. The CaO thickness of both films is identical, but the morphologies encountered after growth are completely different. For CaO grown in molecular oxygen, small grains are clearly visible and are consistent with spotty RHEED and island nucleation and growth. For material grown in water, there is no evidence of individual CaO grains and the step-and-terrace morphology of the underlying GaN is preserved. Individual line scans reveal step heights that are consistent with one half of a unit cell distance along CaO [111], that is, 2.8 Å. Figure 3: Surface topography comparison for CaO films prepared in oxygen and water vapour. ( a ) GaN starting surface, which is populated by growth spirals with 0.26 nm step heights. These spirals initiate around screw dislocations and are consistent with layer-by-layer growth from a supersaturated MOCVD ambient. ( b ) 4.5 nm CaO film grown in molecular oxygen. The AFM resolves clearly the grainy nature of the CaO coating and how the fine grains decorate the underlying GaN steps and terraces; the RMS roughness over a 5×5 μm area is 0.5 nm. ( c ) 4.5 nm CaO film grown with water vapour; all other conditions identical the step and terrace morphology of the GaN is preserved and the RMS roughness over 5×5 μm is 0.3 nm. Full size image Our results can be interpreted initially by the experimental observations of Hacquart et al . who showed that nanoscale cubes of MgO could be immersed in neutral water and converted by an equilibrium dissolution and precipitation process to octahedra [21] . The explanation for this conversion is based on the calculations of Refson, who found that at 0 K, when fully protonated, the lowest energy crystallographic face of MgO switches from {001} to {111} [22] . Surface hydroxylation (which can be considered as similar to a monolayer of Ca(OH) 2 ) occurs during water immersion, thus in an aqueous environment finite solubility leads to a morphology conversion from cubic to octahedral habit. This equilibrium process relies on chemical boundary conditions and a mechanism for mass transport, thus is not beholden to the liquid phase. A related process is known to occur naturally when the mineral periclase (MgO) is formed by the decarbonation of dolomite (the mineral form of MgCa(CO 3 ) 2 ) on contact with magma. In this situation, the locally CO 2 -rich local environment is believed to stabilize the {111} facets [23] . These natural and artificial examples suggest the presence of a ubiquitous process in which control of chemical boundary conditions can be used to stabilize a desired facet. Specific to the current case, if a growing rocksalt film is nucleated with 〈111〉 orientation and grown in an environment that preserves hydrogen termination, smooth layer-by-layer growth is expected. The principle challenge lies in creating a growth environment that can so influence surface energy and film accumulation. Copel et al . reported an experiment where single monolayers of metals on silicon extend layer-by-layer epitaxy in isostructural systems to larger thicknesses by persuading predominantly step-edge nucleation [24] . Here we show that a transient surfactant layer can alter radically the growth habit in highly heterogeneous systems—an unprecedented effect in thin film synthesis. X-ray diffraction measurements were performed to characterize the extent to which surfactant-assisted growth impacts film properties. In the ω -circle, full-width half-maximum values for the {111} CaO reflection were reduced from 0.3° to 0.2°. This effect can be understood by considering that without a surfactant, there are numerous low-angle boundaries that separate the CaO grains visible to AFM. These boundaries are regions of high disorder and can act as secondary nucleation sites that further contribute to the crystalline mosaicity. Estimates of in-plane mosaicity were made by comparisons of azimuthal scans of the {002} CaO reflection. Deposition in water vapour reduces the FWHM values in φ by a factor of two compared with deposition in oxygen, from 3.7° to 1.6°. Though substantial, these line widths are consistent with the 7% lattice mismatch at this oxide–nitride interface and compare favourably to reports of cubic oxide epitaxy on GaN, particularly with respect to in-plane crystallinity [6] , [12] , [25] , [26] . We note that a low-resolution x-ray diffraction configuration was used (crossed beam collimator and receiving slits) to maximize intensity as the films are 25 nm thick. As such, the comparison of oxygen and water is evident, but instrument broadening is on the order of 1° in φ , thus actual in-plane mosaicity is likely substantially smaller. To elucidate the role of surfactants in stabilizing the 2D epitaxial growth of CaO {111} on GaN (0001), ab initio thermodynamics (AIT) [27] , [28] calculations, using density functional theory [29] , [30] , were performed. The general steps in AIT are energy minimization, zero-point energy corrections, and extension to various temperatures and pressures through the chemical potential. Results of these calculations allow for comparison of temperature-, pressure-, and chemical termination-dependent surface-free energies of CaO grown with and without the surfactant, that is, in pure O 2 or H 2 O. The temperature-dependent calculation is a critical component as it provides a means to identify independently the window in processing space that promotes smooth growth, and a variable against which the outcomes of experiment and calculation can be evaluated for self-consistency. The computational experiment evaluated 16 low-index surface configurations. Previous work on CaO [31] , [32] , [33] and MgO [7] , [22] , [31] , [34] , [35] , [36] , [37] , [38] was used to identify a set of configurations that are experimentally manageable and practically relevant. In general, bare relaxed, bare reconstructed, hydrated (associative adsorption of H 2 O), and hydroxylated (dissociative adsorption of H 2 O) surfaces were considered. Table 1 lists the entire set and their primary surface characteristics. Table 1 Surface configurations evaluated with ab initio thermodynamics calculations. 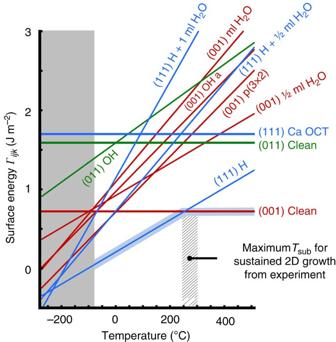Figure 4: Temperature-dependent comparison of relevant CaO surfaces. Surface free energy values as a function of temperature for a collection of relevant CaO surface orientations and chemical terminations involving bulk, bulk reconstructed, hydroxylated and hydrated. The grey region marks the upper limit of the chemical potential. Full size table Figure 4 shows a subset of temperature-dependent surface free energy calculations at a water partial pressure of 5×10 −4 Torr. This pressure was chosen as it represents the best assessment of pressure at the substrate locally, and is based on the report of Theis and Scholm [39] . Not all of the configurations are shown. High-energy surfaces, like the polar bulk facet (111) with Ca or O termination, are not included. The lowest energy for any configuration is highlighted for clarity. It is apparent from the surface free energy plot in Figure 4 that the hydroxylated (111) surface formed during surfactant growth has the lowest surface free energy at this partial pressure up to a temperature of 253 °C. Beyond this temperature, the lowest energy configuration becomes the bare (001) surface. These results provide definitive evidence that the surfactant significantly lowers the surface free energy of the hydroxylated (111) bulk facet as compared with any other surface over a finite range in temperature at a fixed pressure. This preserves the epitaxially preferred habit and prevents the Ca- or O-octopole reconstruction, which would be the energetically preferred (111) habit in the absence of hydrogen in the same temperature regime. It is worth noting that the octopolar reconstruction of the CaO (111) exposes {001} type nano-facets. It is likely that this surface reconstruction provides a pathway to defeat the epitaxial preference for flat (111) growth on GaN (0001) and leads to the rough-growth mode seen experimentally in oxygen. Lowering the surface free energy of the (111) bulk facet by the hydroxyl surfactant prevents this reconstruction from occurring and promotes smooth 2D growth. Figure 4: Temperature-dependent comparison of relevant CaO surfaces. Surface free energy values as a function of temperature for a collection of relevant CaO surface orientations and chemical terminations involving bulk, bulk reconstructed, hydroxylated and hydrated. The grey region marks the upper limit of the chemical potential. Full size image To fully explore the temperature-dependent predictions of AIT calculations, a set of depositions with increasing substrate temperature (all other conditions identical) was conducted to determine the temperature at which the surfactant effect was no longer effective. Assessment of this was based on the number of RHEED oscillations that could be sustained. Depositions were conducted in 50 °C increments. From 150 °C to 450 °C, an increase in oscillations was observed until a maximum of ~35 distinct oscillations were visible at 250 °C. We note that after oscillations subsided, AFM images of surfaces retain the step-and-terrace morphology. At 300 °C, the number of visible oscillations are reduced, and by 400 °C only, several oscillations are observed before complete damping. We therefore identify a temperature in the range of 250 °C to 300 °C as the range above which the surfactant surface becomes unstable. The surface energy calculations predict this situation at 253 °C. This agreement is within the experimental abilities to know substrate temperature and pressure, and the errors associated with simulation results. Though temperature dependent, the sticking coefficient of H 2 O is not the primary factor establishing the window of 2D growth. Two observations support this: at T sub =250°C and p H 2 O=10 −5 Torr, increasing the Ca flux by a factor of three yields no change in time-dependent RHEED oscillations, and CaO grows at temperatures well above the 2D to 3D growth mode transition. The lack of strong flux dependence near the 2D to 3D transition suggests that supply of H 2 O is not a limiting factor, and if the sticking coefficient became small enough to eliminate surface hydroxylation, a transition to Ca metal deposition would be seen as H 2 O is the sole oxidant present. To demonstrate the impact of this approach, beyond a clear improvement in synthesis science, simple planar capacitor structures were prepared on n -type GaN substrates. Preparing gate and passivation oxides on GaN surfaces remains an important challenge, and provides a context in which the value of a smooth CaO morphology can be estimated [40] . The CaO capacitors have a constant dielectric thickness of 4.5 nm and a Dy 2 O 3 cap thickness of 0.8 nm. Metal clips were used to mask a portion of the GaN surface for subsequent bottom contact. Thin structures were selected, because they provide a greater challenge with respect to sensitivity to morphological defects and they represent a capacitance density that is relevant with respect to device needs. The MIS capacitors were completed with Pt electrodes. The band offsets between CaO and GaN were measured previously and conduction barriers to electrons and holes have been identified [41] . 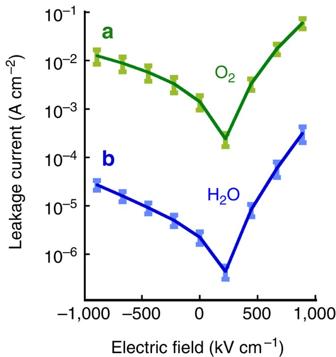Figure 5: Leakage current comparison for CaO films prepared in oxygen and water vapour. Leakage current analysis of 4.5 nm CaO capacitors. (a) Surfactant-assisted CaO plus capping layer. (b) Conventional CaO plus capping layer. Each trace is an average of data captured for 20 capacitors. The error bars correspond to the standard deviation values at each voltage. The offset in field corresponds to 0.1 V and is consistent with the Schottky barrier known to exist at the GaN | CaO interface41. Figure 5 provides the results of leakage current measurements as a function of applied electric field for the two capacitor sets showing clear enhancement of film resistivity for material prepared in the presence of water surfactant. The smooth morphology reduces leakage current density by between 100 and 1,000 times at an equivalent electric field. The lines represent average values for 10 dot capacitors whereas the error bars correspond to the standard deviation within each sample type. Though not reflected by the RMS roughness differences, line scans taken from AFM images of the O 2 -grown material reveal local asperities that are on average 1.5-nm tall. Such undulations are not observed when films are prepared in water vapour. We attribute the contrast in leakage to the presence of these asperities and their ability to locally concentrate the electric field. We note that thickness-dependent XPS studies of CaO growth on GaN in oxygen by Craft et al . revealed that complete surface coverage (as determined by decay of the Ga 2p photoelectron line intensity with overlayer thickness) did not occur until about 1.5 nm of deposition [41] . This value is consistent with the magnitude of the asperities observed by AFM on the present samples. Figure 5: Leakage current comparison for CaO films prepared in oxygen and water vapour. Leakage current analysis of 4.5 nm CaO capacitors. ( a ) Surfactant-assisted CaO plus capping layer. ( b ) Conventional CaO plus capping layer. Each trace is an average of data captured for 20 capacitors. The error bars correspond to the standard deviation values at each voltage. The offset in field corresponds to 0.1 V and is consistent with the Schottky barrier known to exist at the GaN | CaO interface [41] . Full size image It is important to consider the terminal surface composition of material prepared in H 2 O vapour and its impact on properties. Liu et al . reported that CaO crystals exposed to water vapour in comparable pressures to the present study accumulate 0.9 monolayers of hydroxide through a chemical dissociation mechanism. It is sensible to assume that surfactant-assisted CaO films have a similar terminal surface. The impact of this surface on electrical properties is not known directly; however, leakage current densities indicate resistivity values of 10 10 Ω cm at 0.5 MV cm −1 . This range is consistent with wide bandgap insulators and suggests, though indirectly, that hydrogen incorporation in the film bulk is small and that the hydroxide termination does not impart a predominant effect [20] . Surfactant-assisted PVD conquers the morphology barrier to highly heterogeneous epitaxy and presents the field of oxide electronics with new opportunities to traverse obstacles of symmetry and composition with a degree of structural perfection that was, before this time, beyond reach. Our methodology is illustrated for the model system of {111} CaO on (0001) GaN. Under conventional conditions, CaO defaults within a few monolayers to Volmer–Weber growth and rough surfaces. Introducing a water surfactant induces a layer-by-layer mode, for which robust RHEED oscillations are observed in situ . Ab initio thermodynamic calculations predict that in the presence of the surfactant, flat {111} CaO surfaces are stabilized by hydroxylation over a range of temperatures. This surfactant approach introduces a new control variable previously ignored in PVD, namely the chemical boundary condition. Adding surfactants to the existing repertoire of deposition tools of lattice match, energetic bombardment, and shuttered fluxes empowers the thin-film community with an expanded latitude to create artificial heterostructures that lead to new interface science and new technology concepts. Thin film synthesis CaO thin films were grown by oxide MBE using a Perkin-Elmer 435 onto [0001] oriented Ga-face c + -polar films that exhibit a single and uniform polar orientation. Ca was evaporated from an EPI effusion cell filled with Ca pellets (Alfa Aesar 99.99% purity), while the oxidant was supplied as either molecular oxygen or water vapour. A flux of water vapour was produced by connecting, via a controlled UHV variable leak, a stainless steel vessel that was filled with 10 Torr of pure H 2 O vapour, that is, the equilibrium vapour pressure of water at RT. GaN substrates are affixed to a molybdenum puck using a metal clamp. Substrate temperatures are estimated to be 50 °C lower than pyrometric measurements of the Mo pucks, as calibrated by Kumar [42] . GaN films were grown via metal organic chemical vapour deposition onto sapphire substrates with a 20 nm AlN buffer layer. All GaN substrates are silicon-doped ( n -type) Ga-faced and grown to a final thickness of 1.2 μm. The carrier concentration is 3×10 −19 . CaO films were grown using a cell temperature of 465 °C, and substrate temperatures between 150 °C and 450 °C, and a constant growth pressure of 10 −5 Torr O 2 . This pressure is measured with an ion gage located in the back of the growth chamber. Pressure at the substrate surface is ~50-time higher, as calibrated by Theis and Kraisinger, as we introduce both the oxidants via 0.5′-diameter stainless steel tubes confocal to the substrate centre with a tube to substrate distance of 10 cm (ref. 43 ). CaO films were capped with three monolayers of Dy 2 O 3 . Dysprosia caps are grown at the same substrate temperature and growth pressure as the underlying CaO film. Previous studies have shown that these similar growth conditions to CaO also provide high-quality hexagonal 001-Dy 2 O 3 . After CaO deposition, the Ca shutter is closed; the water vapour source is shut off; molecular oxygen is introduced at 10 −5 Torr; and the Dy shutter (Dy cell temperature of 830 °C) is opened. RHEED oscillations are used to determine cap thickness. Thin-film characterization Samples are characterized in-situ using reflection high-energy electron diffraction (RHEED) using a 10-kV beam and a K -space image acquisition system. Samples are characterized ex-situ with atomic force microscopy (AFM) using a Nanosurf Easyscan 2 AFM operated in tapping mode; X-ray diffraction using a Philips X'PERT; and leakage current measurements using a Keithley 617 electrometer. Electrical measurements were collected from MIS-capacitors: contact was made to CaO film with top-Pt electrodes deposited via DC sputtering through a shadow mask, while contact was made to n -GaN substrate with In on the GaN surfaces, underneath the metal clips during CaO deposition. Film thickness for water-grown materials was determined by RHEED oscillations. Thickness measurements for CaO prepared in O 2 were determined by stylus profilometry (Veeco Dektak 150) using films greater than 50 nm to calibrate a growth rate from which films of lower thickness could be prepared. The calibration was performed immediately before electrical property measurement sample preparation to minimize flux drift. CaO films prepared in O 2 show two clear oscillations before island formation. This information was also used to estimate growth rate, and in combination with growth time, was used to predict final thickness. We note that the thicknesses of CaO films for electrical property measurements, when calculated from flux calibration and from the initial RHEED intensity oscillations agree to within 1 CaO monolayer. Computational methods The energies of the CaO systems were calculated using density functional theory as implemented in the Vienna ab initio simulation program [44] , [45] , [46] , [47] . The calculations use the PBEsol refinement [48] to the generalized gradient approximation [49] of the exchange–correlation functional. PBEsol was found in this case to best reproduce bare-surface energies. Hydroxylated surfaces were compared with other exchange correlation potentials, and little variation was found. For each index family considered, the bulk, bare surface, and hydrated and hydroxylated surfaces were calculated in identical periodic simulation cells. The thickness of the surface slabs and vacuum between surfaces was chosen such that their influence would be within the convergence criteria listed below. The kinetic energy cutoff was set to 1,000 eV and the k-point spacing was chosen such that the energy of bulk was converged to within 6.5 meV per atom, and the surface energies to within 4.5 mJ m −2 . For the geometry relaxation, the break condition for the ionic relaxation loop was set to 10 −5 eV. Zero-point energy calculations were performed with the same basis set as the energy calculations, using four displacements in each direction. The total surface free energy of each system was calculated according to equation 1: where γ i,j,k is the energy to create the surface configuration as compared with the original bulk and isolated water when it is present, n is the number of water molecules that adsorb on the surface, μ is the chemical potential of water, a and b are the number of OH groups and water molecules on the surface, respectively, and γ rib are the vibrational contributions to the surface energies. It is assumed that vibrational modes in the bulk cancel. The surface energy, therefore, accounts for the vibrational modes contributed by the surface species only. It also includes a temperature and pressure dependence via the chemical potential of water, which is determined from the JANAF tables [50] . How to cite this article: Paisley, E.A. et al . Surfactant-enabled epitaxy through control of growth mode with chemical boundary conditions. Nat. Commun. 2:461 doi: 10.1038/ncomms1470 (2011).